'Quantized' states of the charge-density wave in microcrystals of K0.3MoO3 Quantization of electrons in solids can typically be observed in microscopic samples if the mean free path of the electrons exceeds the dimensions of the sample. A special case is a quasi one-dimensional metal, in which electrons condense into a collective state. This state, a charge-density wave (CDW), is a periodic modulation of both the lattice and electron density. Here, we demonstrate that samples of K 0.3 MoO 3 , a typical CDW conductor, show jumps in conduction, regular in temperature. The jumps correspond to transitions between discrete states of the CDW and reveal the quantization of the wave vector of electrons near the Fermi vector. The effect involves both quantum and classical features of the CDW: the quantum condensate demonstrates modes, resembling those of a classical wave in a resonator. The analysis of the steps allows extremely precise studies of the CDW wave-vector variations and reveals new prospects for structural studies of electronic crystals and fine effects in their electronic states and lattice motions. The CDW [1] , [2] , [3] , [4] forms as a three-dimensionally (3D) ordered structure below the Peierls transition temperature, T P . Many features peculiar to the CDW are rather vivid and could be illustrated with simple analogies. For example, elastic properties of the CDW can be understood if one conceives it as a three-dimensional electronic crystal inside the host lattice. At the same time, the CDW is a fundamentally quantum object. The CDW wavelength, λ , is close to half the de Broglie wavelength of the Fermi-energy electrons, λ = π / k F . On each conducting chain, the π / k F distortion groups the electrons in pairs and results in an energy gap 2Δ in the electronic spectrum at the Fermi level. Many CDW compounds show metastable states. This means that the CDW can deform; under the effects of an electric field or a temperature change, the wave vector, q ≡2 π /λ, can vary in some allowed range for the given temperature around its equilibrium value, q eq . If the sample ends or the contacts impose tight boundary conditions on the CDW phase, the number of wavelengths in a sample, N , should be integer. So, one can expect 'quantization' of the q -vector in samples of such compounds; there should be a set of discrete states with different integer values of N around N eq at a given temperature, T . 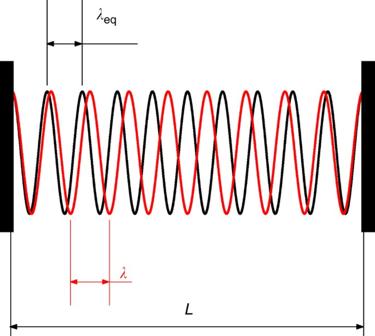Figure 1: Illustration of 'quantization' in a sample with the CDW fixed at the contacts. Suppose the black spring shows the equilibrium state:Neq=10,λeq≡2π/qeq=L/Neq, then the red spring corresponds to a strained CDW:N=9,λ≡2π/q=L/(Neq−1). Typical experimental values are as follows: atT∼100 K for a 30 μm-long sample of K0.3MoO3,Neqis 104, and it can vary by plus/minus several wavelengths. Figure 1 illustrates the 'quantization'. Transitions between the states require local suppression of the CDW state—phase-slip (PS) events. For many CDW compounds, q eq is temperature dependent; hence, an operative way to provoke PS process can be temperature change. Figure 1: Illustration of 'quantization' in a sample with the CDW fixed at the contacts. Suppose the black spring shows the equilibrium state: N eq =10, λ eq ≡2 π / q eq = L / N eq , then the red spring corresponds to a strained CDW: N =9, λ ≡2 π / q = L /( N eq −1). Typical experimental values are as follows: at T ∼ 100 K for a 30 μm-long sample of K 0.3 MoO 3 , N eq is 10 4 , and it can vary by plus/minus several wavelengths. Full size image How does one detect such a PS? Conduction measurements give such a possibility. In fact, the conduction, σ , at an electric fields below the threshold value, E t , is provided by quasiparticles (electrons n and holes p ) excited across the gap. The concentrations n and p simply couple to q variations: a change in q is in a sense equivalent to a change of doping degree [5] . Therefore, in small samples, one can try to resolve transitions between the 'quantized' values of q as step-like changes of the conductivity. In Borodin et al . [6] , Zaitsev-Zotov [7] , Nad' [8] a beautiful size effect, specific only to CDW compounds, has been reported. It has been found that in samples of orthorhombic TaS 3 (o-TaS 3 ), with typical dimensions of 10 × 0.1 × 0.1 μm 3 , the temperature dependences of conduction have an unusual appearance: the σ – T hysteresis loops generated by cooling and then warming are jagged, exhibiting vertical steps directed towards the middle of the loop. The steps were attributed to single PS events between discrete states of the CDW. In fact, according to the estimates [6] , the steps height, δ σ , corresponded, on average, with the creation or annihilation of two electrons per conducting chain, as should be the case for a PS event. Although the steps are likely to reveal PS events, no discrete conducting states that varied regularly with temperature were observed [6] , [7] . In addition, the steps varied in height. The tentative reason given for this was absence of tight boundary conditions for the CDW [6] , [7] , [9] . The area perturbed by a PS event could spread beyond a contact [9] , and one would measure only a fraction of δ σ associated with deformation between the contacts. The value of δ σ could also decrease because of poor transverse coherence of the CDW in TaS 3 . In this case, a PS event could cover only a part of the sample cross-section. The longitudinal coherence length of the CDW, L 2 π , is also important. It does not affect the value of δ σ , if the perturbed area does not spread beyond the contacts; however, if L 2 π is less than the sample length, the jumps would be irregular in temperature, as the phase would slip independently in different parts of the sample. K 0.3 MoO 3 , the blue bronze (BB) [4] , resembles o-TaS 3 in structure. Above T P , one can consider the conducting band to be approximately quarter-filled in both compounds. However, while in TaS 3 , the band carriers are electrons, in BB, conduction is provided by holes (the electronic band is ¾ filled). Therefore, the CDW in BB is formed of holes. As in o-TaS 3 (ref. 1 ), the q -vector in BB decreases [4] , [10] with decreasing T . Unlike fibrous o-TaS 3 , K 0.3 MoO 3 grows as high-quality, grain-boundary-free single crystals. Therefore, one can expect higher transverse coherence of the CDW in this compound. This is justified by relatively high-precision X-ray diffraction measurements available for BB [10] , which resolve the q change down to ∼ 100 K. Tight boundary conditions for the CDW in thin samples might be achieved if the contacts are deposited with the laser ablation technique. This method provides deep (hundreds of Å) penetration of high-energy ions into the sample and creates radiation defects over an even larger depth. The resulting high value of E t under the contacts would prevent spreading of the PS-induced deformation beyond the contact. Here, we report studies of K 0.3 MoO 3 samples with submicron thickness and contact separation on the order of tens of microns. The conduction of such samples reveals the discrete states of the CDW. Switching between the states happens at regular temperature intervals and it results in nearly equal steps of conduction. The distribution of the jumps in temperature provides the q ( T ) dependence corresponding with the X-ray results [10] , and this gives clear evidence that the steps reveal single PS events. The temperature-dependent conduction The sample preparation process is described in the Methods section. 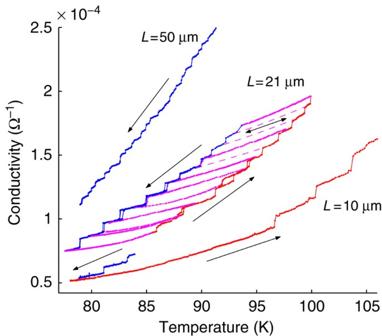Figure 2: Fragments of the temperature dependences of conduction for different samples. The sample dimensions are: 21 × 5 × 0.3 μm3(the representative one), 50 × 7 × 0.3 μm3(σis multiplied by 1.5) and 10 × 2 μm2(σis divided by 1.5). The arrows show the direction of temperature sweeps. The broken lines show the missed reversible fragments of the curves. Figure 2 shows a fragment of σ ( T ) dependence for the representative sample—a rectangular crystal with contact separation L =21 μm ( Supplementary Fig. S1 ). As one can see, the dependence is hysteretic [4] . Both cooling and heating edges of the curve show steps in σ . The jumps are regular in temperature. At higher temperatures, the jumps occur more frequently. The height of the steps is approximately the same; more exactly, they are somewhat smaller on the heating curve. Figure 2: Fragments of the temperature dependences of conduction for different samples. The sample dimensions are: 21 × 5 × 0.3 μm 3 (the representative one), 50 × 7 × 0.3 μm 3 ( σ is multiplied by 1.5) and 10 × 2 μm 2 ( σ is divided by 1.5). The arrows show the direction of temperature sweeps. The broken lines show the missed reversible fragments of the curves. Full size image The steps reveal transitions between discrete states of the CDW. This is clear from the σ ( T ) segments connecting the heating and the cooling edges of the loop. Over these segments, σ ( T ) is reversible . Repeated thermal cycling (and even heating up to room temperature—see Supplementary Fig. S2 ) shows that these curves form a regular structure, and no states can be achieved between them. At the same time, the temperature of switching can slightly fluctuate from cycle to cycle, as should be the case for a thermally activated process [11] . One can see correlation between the density of steps and the contact separation, L . Figure 2 shows fragments of σ ( T ) curves for two other samples, one a factor of 2 shorter (10 μm) and the other 2.5 times longer (50 μm). The number of steps observed in a given temperature interval appears approximately inversely proportional to L (for the longer sample, the steps are not so regular in T ). The steps resemble those obtained for o-TaS 3 (ref. 6 ), although the dimensions of our samples are substantially larger. Moreover, the steps are regular in temperature, nearly equal in value and reveal a set of reproducible discrete states. The step distribution in temperature and the q -vector variation We begin the analysis of the results from the positions of steps in temperature. If each step denotes a single PS event (δ q =±2 π / L ), they can together provide direct information about the wave-vector change without any model assumptions and approximations. In principle, the direction of the q change follows from the direction of the conductivity jumps [6] . Assuming, that q decreases [10] with decreasing T , each step of σ on the cooling curve corresponds to δ N= −1 and δ q= −2 π / L . On the heating curve, the signs of δ N and δ q are positive. Thus, counting the number of steps over a temperature range one obtains the q variation over this range. 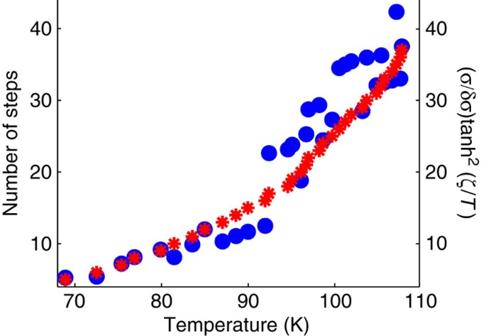Figure 3: The result of steps counting: illustration of the relation between the steps position and height (equation (3)). Stars: Number of steps,m, counted from the lowest temperature (five steps are added as a fitting parameter). Circles:σ/δσ(1−E*/Δ). Both dependences are calculated from the same coolingσ(T) curve for the representative sample. The stars in Figure 3 show the number of steps m obtained from the cooling curve, counted from 69 K to 108 K. Five steps are added to m as a fitting parameter (as discussed below). Multiplying m by 2 π / L , we obtain the change of the q -vector. Figure 3: The result of steps counting: illustration of the relation between the steps position and height (equation (3)). Stars: Number of steps, m , counted from the lowest temperature (five steps are added as a fitting parameter). Circles: σ /δ σ (1− E */Δ). Both dependences are calculated from the same cooling σ ( T ) curve for the representative sample. 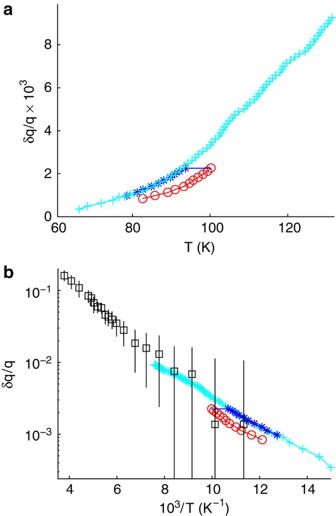Figure 4: The wave-vector variation in BB. (a) δq/qchange for the representative sample calculated fromσ(T) on the assumption that at each step |δq|=2π/L. '+', cooling in a wide temperature range, '*' and 'o', cooling and heating in the narrow temperature range (seeFig. 2). (b) The Arrhenius plot of the same data together with the diffraction results10(squares); the error-bars are also from Giraultet al.10 Full size image Figure 4a shows the temperature variation of the normalized value of the q -vector, δ q / q (0), where q (0)=2 π /[29.7 Å] (ref. 4 ); δ q is reconstructed from counting the steps over a wide-range temperature span ( Supplementary Fig. S3 ) and over the hysteresis loop shown in Figure 2 . Figure 4: The wave-vector variation in BB. ( a ) δ q / q change for the representative sample calculated from σ ( T ) on the assumption that at each step |δ q |=2 π / L . '+', cooling in a wide temperature range, '*' and 'o', cooling and heating in the narrow temperature range (see Fig. 2 ). ( b ) The Arrhenius plot of the same data together with the diffraction results [10] (squares); the error-bars are also from Girault et al . [10] Full size image Previous studies on BB and some other compounds have shown that q ( T ) follows an activation law approaching its T =0 value, with the activation energy close to Δ (ref. 5 ). Figure 4b shows the same data as an Arrhenius plot. With the single-fitting parameter ( Fig. 3 ) δ q (T) represents q ( T )− q (0). Therefore, the five steps that are added to m are the number of PSs, which would reduce q from its value at 69 K down to its zero temperature value. The activation energy, ∼ 500 K, is in good agreement with the known value of Δ: optical reflectivity and photoemission studies give values of Δ between 580 and 870 K (ref. 4 ), and studies of Hall effect give Δ=616 K (ref. 12 ). The results of diffraction studies [10] are also shown in Figure 4b . One can see good agreement between q values obtained from conductivity and diffraction measurements. Surprisingly, the σ ( T ) measurements give much higher resolution in q changes (for example, for a 30 μm sample, one can resolve δ q / q =10 −4 or δ q =2 × 10 −5 Å −1 ). Particularly, we resolve the q variation down to lower temperatures and even the q ( T ) hysteresis. Note that this result is insensitive to inhomogeneous CDW deformations, whereas the latter inevitably broaden the diffraction peaks. Here, we should emphasize that the resolution in q of the quoted diffraction results [10] collected on a rotating anode source is far from the resolution limit of the present synchrotron X-ray techniques. As an example [13] , we can mention the studies of electric-field-induced q -vector variation in NbSe 3 , another typical CDW conductor. The error bar [13] varies between 10 −4 and 10 −5 Å −1 , (δ q / q =1.4 × 10 −3 to 1.4 × 10 −4 ). Hence, we can state that the resolution in q -change based on the steps counting is comparable with that of the up-to-date diffraction methods. Here, we can add that our latest studies of NbSe 3 nanosamples (S.G.Z. and V.Ya.P., unpublished observation) showed that steps on the σ(T) dependence can be resolved for this compound as well. In this case, the resolution in δ q / q is ∼ 3 × 10 −5 , and these steps reveal a weak variation of the q -vector (δ q / q on the order of 10 −4 in the whole temperature range below the lower Peierls transition, that is, below 59 K), which has not yet been observed by the diffraction techniques. The steps' height and the carriers' mobility Interpretation of a step height, δ σ , also gives an insight into the microscopic processes within the CDW, although it requires consideration of the low-field conductivity of BB. The simplest approximation is unipolar conductivity ( n -type for the BB [12] ). Each PS event changes the quasiparticle concentration by (1/ π )δ q =2/ L per conducting chain [5] . Then the specific conductivity step is where μ is the mobility of the electrons; e , the elementary charge; and s 0 , area per chain. At ∼ 90 K, μ =13 cm 2 V −1 s −1 (see ref. 12 ), s 0 =15 A 2 (see ref. 14 ). Then δ σ s =1.32 (Ω cm) −1 . The experimental value is 1 (Ω cm) −1 , in nice agreement with equation (1). Alternatively, from the steps' height, one can find the carriers' mobility, 10 cm 2 V −1 s −1 , consistent with a value of μ obtained from the Hall effect [12] . Relation between the step position and height As both the height and the temperature position of each step couple with the q change, there should be a relation between the steps' position and δ σ . One can recall the equation [6] : The approximation corresponds to unipolar conduction, implying a chemical potential shift from the gap middle, ζ , to be well above T . Note that ( q − q (0))/δ q is just the number of steps, m , counted from T =0, so Together with m , Figure 3 shows temperature dependence of ( σ /δ σ )tanh 2 ( ζ / T ). The correcting factor has been calculated [6] as where E * is the activation energy between the steps ( q =const) and Δ=500 K. One can see nice agreement between the two ways of steps processing (see Methods for more details). The boundary conditions and CDW coherence The discrete conducting states and regular transitions between them argue that the contacts impose tight boundary conditions for the CDW phase, whereas it is nearly free between the contacts. The CDW coherence length, or particularly, the length perturbed by a PS event, can be estimated [9] as 2√[ π (d ζ /d q )/ E t ]. In the unipolar approximation d ζ /d q ≈ T /[ q − q (0)]. With q − q 0 ∼ 3×10 −3 q ( Fig. 4 ) and E t =1.4 V cm −1 (for the representative sample), one obtains L 2 π ≈22 μm. This is close to the separation of the contacts in the representative sample and confirms the CDW coherence over the sample length. Note that the CDW is also coherent over the cross-section: each PS event involves all the chains, evidently through a dislocation climb. Of course, the CDW coherence and the effects of contacts require a more detailed discussion. Here, we just note that the CDW coherence does not imply that the number of wavelengths between the contacts is the same for each chain to atomic-scale accuracy. We have demonstrated discrete states in small crystals of BB. The conductivity measurements allow the resolution of a very small relative change of q , ∼ 10 −4 , at least. The temperature distribution of the jumps reveals the q ( T ) dependence below 100 K and its hysteresis. The results clearly demonstrate 'quantization' of CDW states corresponding to the discrete values of electronic de Broglie wavelengths near k F . The 'quantization' of the CDW wave vector opens new prospects for structural studies of electronic crystals and fine effects in their electronic states and lattice motions, such as interference of two CDWs (as in NbSe 3 , NbS 3 ), incommensurate–commensurate transitions, wave-vector fluctuations, including quantum ones and so on. As an example, we can mention the observation of the weak variation of the q -vectors in NbSe 3 nanosamples (S.G.Z. and V.Ya.P., unpublished observation). Sample preparation and measurement technique The small samples were prepared manually: needle-like lamellas were selected from a high-quality batch synthesized by R.E. Thorne, Cornell University. A mask crossing the sample, usually a Bi 2 Sr 2 CaCu 2 0 x whisker, was tightly glued to the sapphire substrate. Two gold contacts were deposited from laser plasma with ablation method over the ends of each sample, which had the form of a rectangular plate ( Supplementary Fig. S1 ). For deposition, we used laser YAG Nd 3+ in the Q-switch mode. The pulse duration was 7 ns, the energy, 20–40 J cm −2 . The resistance was measured with the usual lock-in technique: small alternate current (AC) (typical frequency 3 Hz, amplitude within 5% of the threshold value) was passed through the sample, and the voltage across the sample was detected by a lock-in amplifier [15] , whereas the AC was used as the reference signal. For measurements of current dependences of the differential resistance (for example, see Supplementary Fig. S4 ), the small AC was overlapped over a slowly varying direct current. Abrupt growth of conductivity above E t ∼ 1 V cm −1 and complete synchronization of the sliding CDW under RF irradiation (the Shapiro steps) give evidence for exceptionally high coherence of the CDW in the samples (see Supplementary Fig. S4 ). Corrections for the unipolar approximation The loop σ( T ) for the representative crystal ( Fig. 2 ) gives a vivid illustration of the electron-hole balance [5] in BB. The value of ζ, that is, the degree of unipolarity, depends both on temperature and on the CDW deformation at fixed temperature. The cooling curve ( Fig. 2 ) corresponds to the q ( T ) decrease; hence, q exceeds the equilibrium values (falling behind it). Correspondingly, n−p =[ q − q (0)]/( πs 0 ) also exceeds the equilibrium value [5] , and the unipolar approximation should work better than that for the heating curve. In fact, ζ is larger in this case, and from the relation [6] δ σ s = eμ δ q tanh( ζ / T )/( πs 0 ), one can see that steps should be higher at the cooling curve, in accordance with Figure 2 . Once the steps are higher over the cooling curve, the slopes of the curves at q =const (the reversible lines in Fig. 2 ) are closer to zero near it. Note, that zero slope ( E * =0) would correspond to completely unipolar conductivity ( ζ > T , n ≫ p ). Quantitatively, one can find ζ (neglecting the temperature dependence of μ ) from the equation (4) (ref. 6 ). The decrease of the step height and growth of E * near the heating curve are consistent with approaching the intrinsic conductivity ( n = p ). Within the cooling curve ( Fig. 2 ), ζ also changes, being grater at lower temperatures than at higher. As an illustration, the smallest E * is ∼ 80 K, and with Δ=500 K, it results in ζ / T =1.6. At the other side of the hysteresis loop, ζ / T= 1.1. This result agrees with the loop width (δ σ / σ ≈δ ζ / T ). The correcting factor, 1− E * /Δ, used for the points in Figure 3 , varies from 0.96 at 69 K to 0.5 at 108 K. Thus, our measurements demonstrate 'quantization' of the CDW also in conductivity. In contrast to the q -value, this 'quantization' is approximate, that is, it requires a correction, as the conductivity is not entirely unipolar. How to cite this article: Zybtsev, S.G. et al . 'Quantized' states of the charge-density wave in microcrystals of K 0.3 MoO 3 . Nat. Commun. 1:85 doi: 10.1038/ncomms1087 (2010).